Escape from crossover interference increases with maternal age Recombination plays a fundamental role in meiosis, ensuring the proper segregation of chromosomes and contributing to genetic diversity by generating novel combinations of alleles. Here, we use data derived from direct-to-consumer genetic testing to investigate patterns of recombination in over 4,200 families. Our analysis reveals a number of sex differences in the distribution of recombination. We find the fraction of male events occurring within hotspots to be 4.6% higher than for females. We confirm that the recombination rate increases with maternal age, while hotspot usage decreases, with no such effects observed in males. Finally, we show that the placement of female recombination events appears to become increasingly deregulated with maternal age, with an increasing fraction of events observed within closer proximity to each other than would be expected under simple models of crossover interference. Recombination is a fundamental meiotic process that is required to ensure the proper segregation of chromosomes. In mammals and other eukaryotes, at least one crossover is normally required to ensure proper disjunction, and failures in recombination can result in deleterious outcomes such as aneuploidy. As such, the recombination process is highly regulated to ensure that sufficient numbers of crossovers occur. The placement of crossover events along a chromosome is also tightly regulated. At the fine scale, the majority of crossovers tend to occur within localized regions of ~2 kb in width known as recombination hotspots. At broader scales, interference between crossovers appears to increase spacing between events occurring on the same chromosome during meiosis. As relatively few crossover events occur within a single meiosis, quantifying the recombination landscape requires the observation of large numbers of meioses. In this study, we adopt a pedigree approach to study the properties of recombination in over 18,000 meioses using data derived from families genotyped via direct-to-consumer genetic testing. Our approach enables hundreds of thousands of recombination events to be localized, and allows us to investigate how the frequency and placement of recombination changes as a function of sex and parental age. To investigate properties of crossover placement in humans, we collected data from pedigree families contained within the database of 23andMe Inc. (Mountain View, CA). Our data set consists of 4,209 families contributing a total of 18,302 informative meioses genotyped at over 515,972 sites. To preserve the privacy of the participants, families were removed if the age of the mother was greater than 40 years at the time of childbirth, the age of the father was greater than 45 years or the difference between the parental ages was greater than 15 years ( Supplementary Fig. 1 ). 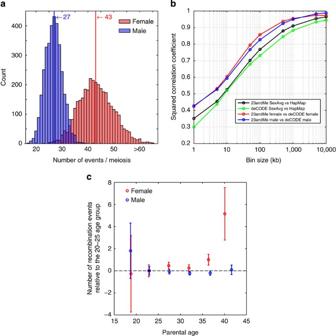Figure 1: Properties of recombination partitioned by sex and age. (a) The number of events per meiosis for females (red,n=9152) and males (blue,n=9150), with median values indicated by a vertical line. For phase-unknown individuals, the average number of events per meiosis was used. (b) Squared Pearson correlation between the 23andMe map, the deCODE map and the HapMap map, as a function of scale. (c) The number of recombination events as a function of parental age for females (red,n=9152) and males (blue,n=9150), relative to parents of between 20 and 25 years of age. Parents were grouped into 5-year age bins, and the mean number of events estimated. Error bars show a 95% confidence interval for each group. 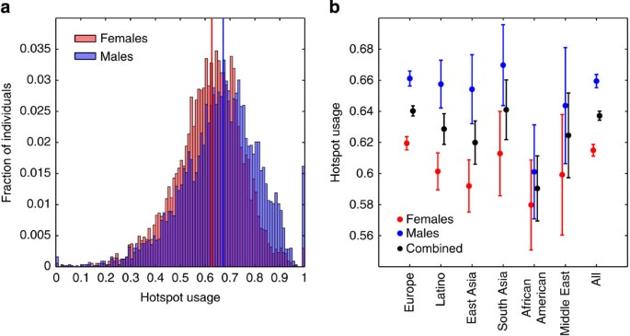Figure 2: Sex differences in recombination hotspot usage. (a) Hotspot usage for female (red,n=9152) and male (blue,n=9150) meioses. Median values for each sex are shown by vertical lines. (b) Mean hotspot usage, subdivided by parental population. Females are shown in red, males in blue and a combined estimate in black. Error bars indicate a 95% confidence interval. The majority of the data is derived from family quartets ( Supplementary Table 1 ), accounting for 78.6% of the families, and is also predominately composed of individuals of European ancestry ( Supplementary Table 2 ). Ancestral populations are assigned to each individual by comparison with a set of reference populations (see Supplementary Methods ). To infer recombination events in nuclear families, we applied the Lander–Green algorithm as implemented within ref. 1 . To guard against genotyping error, we curated the data to remove nearby recombination events that could be indicative of genotyping error (see Supplementary Methods ; Supplementary Fig. 2 ). This approach allowed us to identify over 645,000 well-supported crossover events, with the median event being localized to 28.2 kb ( Supplementary Fig. 3 ). We inferred a mean of 41.6 autosomal recombination events per gamete in females (95% confidence interval (CI): 41.4–41.9) and 26.6 in males (95% CI: 26.5–26.7, Fig. 1a ). The genetic map constructed from our data agrees well with those generated by previous studies ( Fig. 1b ; Supplementary Fig. 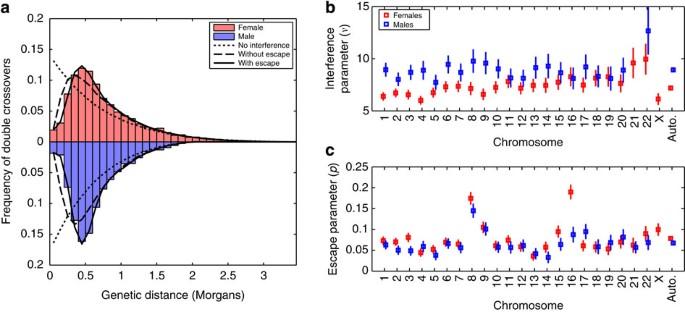Figure 3: Estimation of crossover interference parameters. (a) Fit of three models of interference to the inter-crossover distances observed on chromosome 1, derived from phase-known mothers (red,n=2184) and fathers (blue,n=2092). The interference-free model is shown as a dotted line, the gamma simple interference model is shown as a dashed line and the Housworth–Stahl interference escape model is shown as a solid line. (b) Per-chromosome estimates of the interference parameter as estimated from the Housworth–Stahl interference escape model. Error bars indicate a 95% confidence interval. Note that chr21 in males is excluded due to an extremely high estimate. (c) Per-chromosome estimates of the proportion of events escaping interference. Error bars indicate a 95% confidence interval. 4 ; Supplementary Table 3 ). At the 5-Mb scale, the Pearson correlation between our map and that of deCODE [2] is r 2 =0.975 and 0.983 for females and males, respectively. Likewise, our sex-averaged map has a correlation of r 2 =0.955 with the HapMap map inferred from patterns of linkage disequilibrium (LD) [3] . At the chromosome scale, the map length is well predicated by the physical chromosome length ( r 2 =0.991 in females and 0.945 in males; Supplementary Fig. 5 ). Figure 1: Properties of recombination partitioned by sex and age. ( a ) The number of events per meiosis for females (red, n =9152) and males (blue, n =9150), with median values indicated by a vertical line. For phase-unknown individuals, the average number of events per meiosis was used. ( b ) Squared Pearson correlation between the 23andMe map, the deCODE map and the HapMap map, as a function of scale. ( c ) The number of recombination events as a function of parental age for females (red, n =9152) and males (blue, n =9150), relative to parents of between 20 and 25 years of age. Parents were grouped into 5-year age bins, and the mean number of events estimated. Error bars show a 95% confidence interval for each group. Full size image Treating the overall recombination rate as a phenotype, we replicate genetic associations at genome-wide significance for RNF212, which is known to be essential for crossover-specific complexes [4] , and within the vicinity of TTC5, which appears to replicate an association with CCNB1IP1 (ref. 5 ). 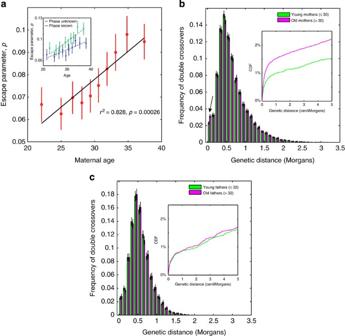Figure 4: Departures from simple crossover interference. (a) Inferred escape parameter as a function of maternal age. Mothers were divided into 10 approximately equal-sized deciles on the basis of age, and the Housworth–Stahl interference escape model was fitted for each group separately. The inset shows the estimates of the escape parameter when considering phase-known (blue,n=2184) and phase-unknown (green,n=6968) individuals separately. Estimates for ν show no correlation with age (Supplementary Fig. 9). Error bars indicate 95% confidence intervals. (b) Distribution of inter-crossover distances for young and old mothers, where the boundary between young and old is taken as median maternal age (30 years). Error bars represent a 95% confidence interval assessed via 1000 bootstrap samples, and the arrow highlights a significant difference between the young and old groups for tightly clustered events. The inset shows the cumulative distribution function (CDF) up to 5 cM. (c) Distribution of inter-crossover distances for young and old fathers, where the boundary between young and old is taken as median paternal age (32 years). Another association near SMEK1 also replicates discoveries elsewhere [5] , but not at genome-wide significance ( Supplementary Table 4 ). Previous reports have suggested increased recombination rates in older females [6] , [7] . Using linear regression ( Supplementary Fig. 6 ), we obtain a similar result with an additional 0.067 events per year being observed in females ( P =0.002, F -test), and no such effect being observed in males ( P =0.30, F -test). The female effect appears to be driven by sharp increase in the number of recombination events for older mothers ( Fig. 1c ). Fitting the piecewise-linear model with a single change point infers a rapid increase in the female recombination rate after 38.8 years, increasing from 0.047 events per year to 2.990 events per year. On average, mothers of 39 years and over have an additional 2.51 events compared with younger mothers ( P =0.0005, Mann–Whitney U ). One possible interpretation of the increasing number of recombination events with maternal age is that mothers with higher recombination rates can maintain fertility until a later age [6] . To investigate this possibility, we focused on 776 mothers (providing 2,184 meioses) that were part of larger families and could have recombination events assigned to specific children. After subtracting off the average age and average number of recombination events for each mother, the resulting regression does not find a significant association with age ( P =0.11, F -test), although we estimate our power to detect an effect size of an additional 0.067 events per year in this subsample to be no more than 30%. Both pedigree and LD studies have suggested that ~60–70% of crossover events occur within recombination hotspots [7] , [8] . Our data confirm this result with 62.7% of events occurring within LD-defined hotspots in females, and 67.3% occurring within hotspots in males ( Fig. 2a ; Supplementary Fig. 7A ). The 4.6% difference between the two sexes is highly significant ( P =1.1 × 10 −69 , Mann–Whitney U ), suggesting differences in the regulation of crossover placement between the sexes. The result remains significant after thinning the female data to match the crossover density of the male data ( P <2.2 × 10 −16 , Mann–Whitney U ), and does not appear to be driven by increased male recombination rates near the telomeres (see Supplementary Methods ). Figure 2: Sex differences in recombination hotspot usage. ( a ) Hotspot usage for female (red, n =9152) and male (blue, n =9150) meioses. Median values for each sex are shown by vertical lines. ( b ) Mean hotspot usage, subdivided by parental population. Females are shown in red, males in blue and a combined estimate in black. Error bars indicate a 95% confidence interval. Full size image Hotspot localization is believed to be under the control of the zinc-finger protein PRDM9, which recognizes and binds specific DNA motifs [9] , [10] , [11] . We find single-nucleotide polymorphisms (SNPs) in the vicinity of PRDM9 to be strongly associated with the degree of hotspot usage, as has previously been reported [5] , [11] . The most strongly associated SNP is rs73742307 achieving a P value of 7.9 × 10 −184 (ref. 4 ), with no other region achieving a genome-wide significant association with this phenotype ( Supplementary Table 5 ). Variation within the PRDM9 DNA-binding domain can result in changes to the recognized motif and hence lead to differences in hotspot localization between individuals. While the major allele of PRDM9 (allele A) is present at high frequency in most human populations, a large number of low-frequency alleles have been observed, particularly within African populations [10] , [12] . Consistent with this, we find hotspot usage to be significantly lower within individuals of African ancestry ( Fig. 2b ; Supplementary Table 6 ), which reflects the fact that the LD-defined hotspots are expected to mostly represent the common PRDM9 allele. Notably, while over 75% of our data are derived from individuals of European ancestry, hotspot usage is higher for males than females across all ancestries. We find a weak association between hotspot usage and maternal age ( Supplementary Fig. 7B ). Using logistic regression, we estimate a decrease in hotspot usage corresponding to ~1% over a 10-year period ( β 1 =−0.0042, s.e.=9.6 × 10 −4 , P =1.2 × 10 −5 , F -test). To ensure this effect is not driven by differences in parental ancestry within the sample, we repeated the analysis only using individuals of European ancestry. In this case, the effect size remains similar ( β 1 =−0.0033, s.e.=0.0013), but is only marginally significant ( P =0.0101, F -test). Including the number of events as an additional predictor variable within the regression leaves age as a weakly significant predictor ( P =0.0106, F -test), but not the number of events ( P =0.74, F -test). Despite the small size of the estimated effect, we note that no such age-related effects were observed in males. To learn more about interactions between recombination events, we used the high number of crossover locations in our data to better characterize the phenomenon of crossover interference. By considering the distribution inter-crossover distances, we fit three models to describe the distribution of inter-crossover distances: a model without interference between crossovers (also known as the gamma model of crossover interference [13] ), and a mixture model in which a subset of events come from a process that exhibits no interference (also known as the Housworth–Stahl model [14] ). To fit these models, we used existing methods for families in which recombination events could be assigned to specific individuals, and extended these methods for smaller families where recombination events cannot be simply assigned to a specific individual (see Supplementary Methods ). In agreement with previous reports [14] , [15] , the Housworth–Stahl interference escape model provides a much better fit to our data than either the gamma simple interference model or the interference-free model ( Fig. 3a ). Under this model, the estimates of the strength of crossover interference are similar to previous reported using smaller data sets [15] . The degree of interference is inferred to be lower in females than in males ( ν female =7.19 vs ν male =8.93). In addition, 7.8%/6.7% of female/male events are inferred to escape interference. We therefore conclude that a non-negligible fraction of crossovers occur in the absence of crossover interference. Figure 3: Estimation of crossover interference parameters. ( a ) Fit of three models of interference to the inter-crossover distances observed on chromosome 1, derived from phase-known mothers (red, n =2184) and fathers (blue, n =2092). The interference-free model is shown as a dotted line, the gamma simple interference model is shown as a dashed line and the Housworth–Stahl interference escape model is shown as a solid line. ( b ) Per-chromosome estimates of the interference parameter as estimated from the Housworth–Stahl interference escape model. Error bars indicate a 95% confidence interval. Note that chr21 in males is excluded due to an extremely high estimate. ( c ) Per-chromosome estimates of the proportion of events escaping interference. Error bars indicate a 95% confidence interval. Full size image We find evidence that both the degree of interference and interference escape varies across chromosomes ( Fig. 3b,c ; Supplementary Table 7 ). The strength of interference is reasonably well predicted by the chromosome map length ( r 2 =0.565, P =6.4 × 10 −9 ), although the relationship is only significant in females when considering the sexes separately ( r 2 female =0.69, P =1.7 × 10 −6 and r 2 male =0.172, P =0.06; Supplementary Fig. 8 ). In contrast, the fraction of events escaping interference shows no relationship with chromosome map length ( r 2 =0.001, P =0.84). Certain chromosomes appear to have high degrees of escape, with chromosomes 8, 9 and 16 (in females) being notable outliers. To investigate whether crossover interference changes with parental age, we subdivided our data into 10 quantiles on the basis of age, and fit the Housworth–Stahl interference escape model to each group independently. We observe a striking increase in the proportion of events that escape interference with maternal age ( Fig. 4a ), rising from 6.7% for mothers under 25 years to 9.5% for mothers over 35 years. No such correlation is observed for the interference parameter in females, and no correlation is observed for either parameter in males ( Supplementary Fig. 9 ). The effect is robust different subdivisions of the data ( Supplementary Figs 10 and 11 ). Figure 4: Departures from simple crossover interference. ( a ) Inferred escape parameter as a function of maternal age. Mothers were divided into 10 approximately equal-sized deciles on the basis of age, and the Housworth–Stahl interference escape model was fitted for each group separately. The inset shows the estimates of the escape parameter when considering phase-known (blue, n =2184) and phase-unknown (green, n =6968) individuals separately. Estimates for ν show no correlation with age ( Supplementary Fig. 9 ). Error bars indicate 95% confidence intervals. ( b ) Distribution of inter-crossover distances for young and old mothers, where the boundary between young and old is taken as median maternal age (30 years). Error bars represent a 95% confidence interval assessed via 1000 bootstrap samples, and the arrow highlights a significant difference between the young and old groups for tightly clustered events. The inset shows the cumulative distribution function (CDF) up to 5 cM. ( c ) Distribution of inter-crossover distances for young and old fathers, where the boundary between young and old is taken as median paternal age (32 years). Full size image A potential concern is that the detected increase in interference escape could be driven by the observed increased number of crossovers in older mothers. If the number of crossovers is increased, then the distances between them are necessarily shorter, which may in turn influence the interference parameter estimates. To account for this possibility, we performed stratified sampling of individuals to control for the number of events within each quantile. The observed increase in the escape parameter with maternal age is still observed ( Supplementary Fig. 12 ), indicating that it is not driven by changes in the overall recombination rate. To further investigate the differences between old and young parents, we plotted the distribution of inter-crossover distances for young and old parents ( Fig. 4b,c ). The interference escape effect in females appears to be predominately driven by an increase in the number of very tightly clustered events, generally separated by less than ~5 cM. These tightly clustered events are not well captured by the Housworth–Stahl interference escape model ( Supplementary Fig. 13 ), and a major concern therefore is that these tightly clustered events represent false-positive calls arising from genotyping error. However, the effect remains even if we apply much stricter filtering of the crossover events ( Supplementary Fig. 14 ), and in addition we believe genotyping error is unlikely to explain the association between the escape parameter and maternal age because (a) the effect is not seen in males, and (b) it would imply increased genotyping error for older mothers (but not fathers). In terms of meiosis, a major difference between the sexes is that female meiosis starts during fetal development, but does not complete until adulthood. As such, while male gametes are produced throughout adulthood and promptly proceed through meiosis, oocytes remain arrested in a late stage of prophase (dictyotene) for many years, if not decades. Presuming our observation of increasing crossover interference escape with maternal age is not due to some obscure form of genotyping error, our observations add to similar evidence of increasing rates of recombination [6] and aneuploidy [16] in aging females. Although these phenomena are presumably related, the biological mechanisms by which they occur are unclear, and we can think of at least three possibilities. First, given chromatids remain physically proximal during the extended period of female meiotic arrest, one possible explanation is that additional recombinations are initiated during this time, perhaps in response to DNA damage. However, as recombination is believed to have completed by the time of dictyotene, such an explanation appears unlikely. A second possibility, previously invoked to explain the increasing recombination rate with maternal age [6] , suggests oocytes with additional recombination events could be at reduced risk of nondisjunction, and hence would be more likely to lead to viable embryos in older mothers. However, it is not clear that this mechanism would explain the increased clustering of events observed in our data. Finally, a third possibility is related to the so-called ‘production line’ hypothesis, in which oocytes are selected for maturation sequentially in the same order as their generation, and later oocytes have therefore potentially undergone additional mitotic divisions prior to entering meiosis [17] . However, the existence of a production line has been debated for many years [17] , [18] , [19] , and so the likelihood of this explanation is unclear. Sample genotyping Samples were collected and genotyped at the consumer genetics company 23andMe Inc., as described previously [20] . Briefly, genotyping was performed on genomic DNA extracted from saliva samples. DNA was genotyped on one of two microarray platforms: the Illumina HumanHap550+BeadChip platform, which includes more than 550,000 SNPs, or the Illumina HumanOmniExpress+BeadChip, which has a base set of 730,000 SNPs augmented with ~250,000 SNPs to obtain a superset of the HumanHap550+, as well as a custom set of about 30,000 SNPs. Pedigree construction Pedigrees were constructed first by identifying trios using estimated identity-by-decent relationships. Trios were then combined to form nuclear families, and nuclear families were joined based on the assumed relationships to form larger pedigrees. We identified trios by finding triplets of individuals in the 23andMe customer cohort that had estimated identity-by-decent relationships matching those expected in a true trio. Trios were accepted if both parents were at least 18 years old upon the birth of the child and one parent was male and the other female. We created nuclear families by identifying all trios with the same two parents and then by combining the children of these trios. Finally, larger pedigrees were created by simply joining the nuclear families based on the assumed relationships and by accounting for directionality given by the age of individuals. Any two individuals with more than one potential relationship were excluded along with the pedigrees they belonged to. Calling of recombination events and data filtering Prior to data filtering, the data set consisted of 4,270 pedigree families, with data pertaining to 18,647 informative meioses. This raw data set consisted of 692,876 recombination events, with a median of 45 and 28 events per meiosis in females and males, respectively. The Merlin algorithm (version 1.1.2) used to detect recombination events does not account for genotyping error, and genotyping errors are therefore likely to result in spurious recombination event calls. To account for this issue, our first step was to only use high-confidence sites. First, we required the sites to have a call rate greater than 90% and Hardy–Weinberg P value ≤1 × 10 −20 (as calculated in the 23andMe cohort). Second, we excluded sites with minor allele frequencies differing from those of the 1000 Genomes Phase 1 reference panel [21] . This was achieved by constructing a 2 × 2 contingency table and comparing the 1000 Genomes European allele counts with those from 2,000 randomly selection 23andMe customers, and using a χ 2 -test to identify significant deviations. Sites with P values less than 1 × 10 −15 were removed. Having applied these basic site filters, we next aimed to remove any weakly supported recombination events. This was achieved by first using the Merlin ‘error’ feature to remove potential genotyping errors not consistent with gene flow within each pedigree. In addition, we excluded all recombination events supported by less than three recombination-informative sites on either side, where we define an informative site as a site that is called as heterozygotic in exactly two individuals out of each mother–father–child trio. Finally, we removed all pairs of events within each single family that occurred within the same SNP interval. Together, these filters removed 31,742 weakly supported events, which corresponded to 4.6% of the total number. Preliminary inspection of the genetic maps identified a region on chromosome 10 where the 23andMe genetic map diverged substantially from that generated by deCODE [2] . This can be seen in a plot of the chromosome 10 genetic map at ~50 Mb ( Supplementary Fig. 2A ). Further investigation of this region revealed a large number of ‘double’ crossovers in close proximity to each other (that is, pairs of recombination events occurring in close proximity within the same individual). While some such observations are expected through the action of gene conversion, such strong clustering of these events is not expected biologically. Instead, we believe the result is suggestive of misplacement of polymorphisms, mis-assembly of one or more reference contigs in the hg19 reference genome or of more complex types of error related to copy number polymorphism or array design. In any case, these double-recombination events represent a form of error that needed to be eliminated. To better quantify this issue, we identified all pairs of recombination events occurring within a single individual that were within 1 Mb of each other. For each SNP in the genome, we estimated the number of these event pairs that span the SNP ( Supplementary Fig. 2B ). For the vast majority of the genome, there were very few such event pairs, and hence localized peaks likely represent data quality issues. We therefore identified all SNPs spanned by at least than 14 event pairs (with this threshold being equivalent to the 99.9th percentile of the distribution). In this way, we identified 50 regions with strong enrichment of nearby event pairs ( Supplementary Table 8 ). Note that for this analysis we ignored the pseudoautosome, as a large number of events occurring in close proximity might be expected due to the extreme male recombination rate within this region. The regions with high numbers of clustered events were themselves clustered into 13 regions across 8 chromosomes, and are often in the vicinity of chromosome centromeres, telomeres or reference assembly gaps. We removed all event pairs within 500 kb of the region boundaries described in Supplementary Table 8 , which resulted in the removal of 2,916 events (0.42% of the total). The removal of these events improved the concordance between the 23andMe and deCODE maps ( Supplementary Fig. 2C ). Previous research using well-curated data in 728 meioses reported an average of 39.6 autosomal events per gamete in females (95% CI 38.5–40.6), and 26.2 autosomal events per gamete in males (95% CI 25.6–26.7) [7] . The minimum/maximum number of observed autosomal events in any given meiosis in this data was 19/71 for females, and 16/43 for males (Graham Coop, personal communication). Preliminary analysis of our data revealed a small subset of individuals had biologically unrealistic numbers of recombination events. Our first filtering step was to remove the pedigrees containing these individuals. Specifically, we removed individuals (and their containing pedigrees) that were more than 5 s.d. from the (sex specific) median number of recombination events. To guard against outliers, we used a robust estimate of the s.d. taken as σ =1.4826 MAD, where MAD represents the median absolute deviation. Before filtering, the median number of recombination events was 43 and 27 for females and males, respectively (including chrX and the pseudoautosome). Using the ±5 σ thresholds, we removed pedigrees containing any female with fewer than 10 or more than 76 events per meiosis, or any male with fewer than 9 or more than 45 events. These filters removed a total of 52 pedigrees. Summary of the filtered data set After applying the filtering steps described above, the filtered data set consists of 4,209 pedigrees containing 18,302 informative meioses, of which 9,152 are from females and 9,150 are from males. Of the families included in the study, 78.6% are family quartets, 14.3% are larger one-generation families, and 7.1% are two-generation families ( Supplementary Table 1 ). Due to the structure of the pedigrees included in the study, certain recombination events can be identified as having occurred within a specific child, whereas others cannot. For example, in family quartets, it is generally unclear which child has the recombinant haplotype, and we therefore refer to these events as ‘phase unknown’. Conversely, the child containing the recombinant haplotype can generally be identified in larger pedigree families in which the parental haplotype can be confidently phased, and we therefore refer to these events as ‘phase known’. In total, 4,276 meioses are derived from phase-known individuals, whereas 14,026 are derived from phase-unknown individuals. Of the female meioses, 2,184 are derived from phase-known mothers and 6,968 are from phase-unknown mothers. Of the male meioses, 2,092 are derived from phase-known fathers, and 7,058 are derived from phase-unknown fathers. Individuals were assigned to high-level population groups via comparison with a set of reference populations (see Supplementary Methods ). The majority of individuals in the data set are of European descent, with ~78% of the meioses in the sample occurring within a European individual ( Supplementary Table 2 ). The parental age distribution for the filtered data set is shown in Supplementary Fig. 1 . The mean age was 30 years for females, and 32 for males. The final filtered data set consists of 645,853 recombination events. Including the sex chromosomes, the mean number of recombination events was 43.47 for females ( σ =6.64, 95% CI 43.25–43.69), and 27.04 for males ( σ =3.28, 95% CI 26.94–27.16). For the autosomes alone, the mean number of recombination events was 41.64 for females ( σ =6.34, 95% CI 41.43–41.85) and 26.61 for males ( σ =3.26, 95% CI 26.51–26.73). The distribution of interval sizes to which crossovers could be resolved (that is, the distance between informative markers on either side of the recombination event) is given in Supplementary Fig. 3 . Crossovers could be resolved within a median distance of 28.2 kb. How to cite this article : Campbell, C. L. et al . Escape from crossover interference increases with maternal age. Nat. Commun. 6:6260 doi: 10.1038/ncomms7260 (2015).